In vivomodel with targeted cAMP biosensor reveals changes in receptor–microdomain communication in cardiac disease 3′,5′-cyclic adenosine monophosphate (cAMP) is an ubiquitous second messenger that regulates physiological functions by acting in distinct subcellular microdomains. Although several targeted cAMP biosensors are developed and used in single cells, it is unclear whether such biosensors can be successfully applied in vivo , especially in the context of disease. Here, we describe a transgenic mouse model expressing a targeted cAMP sensor and analyse microdomain-specific second messenger dynamics in the vicinity of the sarcoplasmic/endoplasmic reticulum calcium ATPase (SERCA). We demonstrate the biocompatibility of this targeted sensor and its potential for real-time monitoring of compartmentalized cAMP signalling in adult cardiomyocytes isolated from a healthy mouse heart and from an in vivo cardiac disease model. In particular, we uncover the existence of a phosphodiesterase-dependent receptor–microdomain communication, which is affected in hypertrophy, resulting in reduced β-adrenergic receptor-cAMP signalling to SERCA. 3′,5′-Cyclic adenosine monophosphate (cAMP) is an ubiquitous intracellular second messenger that, by acting in discrete subcellular microdomains, regulates a plethora of physiological and pathological processes including cardiac function and disease [1] , [2] , [3] . This is achieved primarily by cAMP-dependent protein kinase (PKA)-mediated phosphorylation of several proteins involved in calcium handling and excitation–contraction coupling such as L -type calcium channels, ryanodine receptors, troponin I and phospholamban (PLN) [4] . PLN is a small protein regulator of the cardiac sarcoplasmic/endoplasmic reticulum (SR) calcium ATPase 2a (SERCA2a), and upon PKA-dependent phosphorylation, the PLN-mediated SERCA2a inhibition is relieved, leading to an increased diastolic SR calcium reuptake [5] . Over the last three decades, it has been shown that one second messenger cAMP can engage in many different yet specific functional responses, which depend on the nature of extracellular stimulus [6] . This led to the hypothesis that cAMP signalling is organized in the so-called microdomains, which are characterized by a specific composition of receptors, cAMP hydrolysing enzymes phosphodiesterases (PDEs), phosphatases, PKA and its anchoring proteins [3] , [6] , [7] , [8] . PDEs are crucial for negatively regulating cAMP levels and thus for the control of the individual local cAMP signalling events. At least five PDE families (PDE1–4 and 8) are expressed in the heart and can rapidly hydrolyse cAMP to AMP, thereby creating multiple contiguous cAMP microdomains [1] , [9] , [10] , [11] , [12] . This enables the specificity of each cAMP response associated with local pools of PKA responsible for phosphorylation of particular downstream effectors. In cardiomyocytes (CMs), the existence of several cAMP microdomains has been proposed, which are located, for example, around calcium-handling proteins [1] , [13] . Although several localized cAMP biosensors have been developed and used in transfected cell lines or neonatal cardiac cells [14] , it is unclear whether such targeted biosensors can be successfully used in vivo . Since cardiac diseases are associated with abnormal calcium cycling, for example, due to decreased SERCA2a expression and activity [15] , the use of in vivo models would be especially advantageous to study the role of local, microdomain-specific cAMP signalling under cardiac disease conditions. Here, we generated a new targeted Förster resonance energy transfer (FRET)-based biosensor Epac1-PLN and expressed it in transgenic (TG) mice to directly monitor subcellular cAMP dynamics in the SERCA2a microdomain of adult ventricular CMs isolated from healthy and diseased hearts. This approach revealed the biocompatibility of a targeted cAMP biosensor and its usefulness for in vivo cardiac disease models. Furthermore, we uncovered the existence of a privileged receptor–microdomain communication, which is remarkably affected in cardiac disease. Generation of targeted biosensors and TG mice To enable real-time measurements of cAMP dynamics in the SERCA2a microdomain, we sought to develop a biosensor that would report changes of local cAMP levels with high sensitivity in a physiologically relevant context. Therefore, we fused the sequence of the highly sensitive sensor Epac1-camps (effector concentration for half-maximum response for cAMP ∼ 2 μM) [14] , [16] to the N-terminus of PLN. Initially, we generated an analogue of the previously developed SR-ICUE3 biosensor (effector concentration for half-maximum response for cAMP ∼ 15 μM), which lacks the PLN N-terminal cytosolic helix (PLNΔ1-18) involved in pentamer formation and kinase-dependent regulation [17] . However, when tested in transiently transfected 293A cells, such a sensor showed only relatively small changes in FRET upon β-adrenergic stimulation ( Supplementary Fig. 1a–c ). To improve the FRET response and retain normal biochemical properties of PLN, we next developed a construct in which the sensor is fused to the full-length PLN sequence via a flexible linker. This resultant new biosensor called Epac1-PLN showed significantly larger responses. However, since PLN forms pentamers that may rearrange upon PKA-mediated phosphorylation, we sought to study whether these processes may affect FRET responses measured by the Epac1-PLN sensor. To do so, we introduced the previously characterized R279E mutation, which renders the sensor insensitive to cAMP [18] . Importantly, this mutant construct did not show any change in FRET upon β-adrenergic stimulation ( Supplementary Fig. 1b,c ), suggesting that the responses recorded by the Epac1-PLN sensor are exclusively due to cAMP binding. Likewise, co-transfection of sensor constructs with either non-fluorescent donor or acceptor proteins and subsequent measurements showed that the potential change of intermolecular FRET upon cAMP/PKA pathway activation is not likely to significantly contribute to the measured signals ( Supplementary Fig. 1a–d ). Conversely, PKA inhibition with H89 did not change the kinetics and the amplitudes of the FRET responses, ruling out possible contribution of the PKA-dependent sensor phosphorylation to FRET signals ( Supplementary Fig. 1b,c ). Therefore, Epac1-PLN sensor has passed important validation and characterization steps and was used in further experiments. To study cAMP dynamics in the context of in vivo disease models and in freshly isolated adult mouse ventricular CMs, we generated TG mice by pronuclear injection of a construct expressing Epac1-PLN under the control of the α-myosin heavy chain (α-MHC) promoter ( Fig. 1a ). We obtained two mouse lines one of which showed good breeding performance, sensor expression in virtually all cardiomyocytes and its proper localization to the SERCA2a compartment in heart cross-sections of the offspring line ( Fig. 1b ). Isolated TG CMs reacted to the β-adrenergic receptor (β-AR) agonist isoproterenol (ISO) with a clear increase of the CFP/YFP ratio, indicative of an increase in local microdomain cAMP levels ( Fig. 1c ). Morphometric and histological analysis revealed no changes in cardiac morphology, heart-to-body-weight ratios and cell size of TG compared with wildtype (WT) hearts and cells ( Supplementary Fig. 2 ). 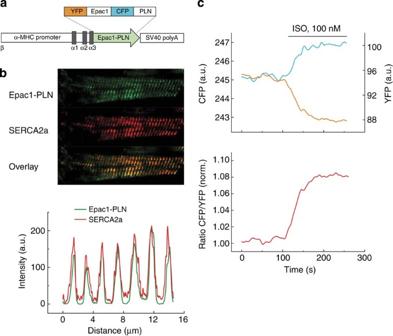Figure 1: Generation of Epac1-PLN transgenic mice. (a) Schematic representation of the Epac1-PLN sensor construct that includes two fluorophores, yellow (YFP) and cyan fluorescent proteins (CFP) flanking the cAMP-binding domain from Epac1 and coupled to phospholamban (PLN). Epac1-PLN was transgenically expressed under the control of the cardiomyocyte-specific α-MHC promoter. (b) Representative confocal image (n>10) of immunostained transgenic Epac1-PLN heart cross-section. Epac1-PLN and SERCA2a co-localization is confirmed by the intensity overlay of both fluorescent signals. (c) Representative single YFP and CFP intensities and CFP/YFP ratio (n>15) of Epac1-PLN cardiomyocytes upon stimulation with isoproterenol (ISO). An increase in the FRET ratio represents an increase in local cAMP. The in vivo heart dimensions and function analysed by echocardiography was not markedly altered, apart from a slight but clearly detectable, significant increase in contractility in TG hearts ( Supplementary Table 1 ). Figure 1: Generation of Epac1-PLN transgenic mice. ( a ) Schematic representation of the Epac1-PLN sensor construct that includes two fluorophores, yellow (YFP) and cyan fluorescent proteins (CFP) flanking the cAMP-binding domain from Epac1 and coupled to phospholamban (PLN). Epac1-PLN was transgenically expressed under the control of the cardiomyocyte-specific α-MHC promoter. ( b ) Representative confocal image ( n >10) of immunostained transgenic Epac1-PLN heart cross-section. Epac1-PLN and SERCA2a co-localization is confirmed by the intensity overlay of both fluorescent signals. ( c ) Representative single YFP and CFP intensities and CFP/YFP ratio ( n >15) of Epac1-PLN cardiomyocytes upon stimulation with isoproterenol (ISO). An increase in the FRET ratio represents an increase in local cAMP. Full size image In CM lysates, Epac1-PLN sensor was detected solely in the SERCA2a-positive membrane fraction ( Supplementary Fig. 3 ), further corroborating the proper sensor localization. Quantitative real-time PCR revealed twofold overexpression of PLN in Epac1-PLN hearts, while the SERCA2a expression analysed by immunoblot was also increased, ultimately leading to an unchanged PLN/SERCA2a ratio ( Supplementary Fig. 4a–d ), which might represent a compensatory mechanism to counterbalance the increase of PLN expression due to Epac1-PLN. Calcium imaging showed almost unaltered calcium decline kinetics in the absence and presence of ISO stimulation, as well as unchanged SR calcium load ( Supplementary Fig. 4e,f ) and calcium transient amplitudes (F 340 /F 380 1.46±0.04 for WT and 1.38±0.04 for TG, means±s.e., P =0.1). Similar to endogenous PLN, Epac1-PLN (monomer ∼ 72 kDa) was also able to form oligomeric complexes and be phosphorylated by PKA at Ser16 ( Supplementary Fig. 5a,b ). Finally, we used gene arrays to verify that the messenger RNA (mRNA) expression levels of the main players involved in cAMP signalling such as β-ARs, G-proteins, adenylyl cyclases, PKAs, PDEs and Epac were not significantly changed between TG and WT cardiomyocytes ( Supplementary Fig. 6 ). Some of these proteins (PKA regulatory subunits, PDE2A and PDE4D8) were also verified in immunoblots using available antibodies ( Supplementary Fig. 7 ). These data strongly suggest that in TG CMs, the molecular composition and the function of the SERCA2a microdomain is preserved and should allow reliable measurements of local cAMP dynamics. Local PDE effects in β 1 -AR-SERCA2a communication Next, we performed FRET recordings under selective stimulations of β 1 - and β 2 -AR in Epac1-PLN-expressing cardiomyocytes and compared local cAMP responses with those measured in the bulk cytosol by using previously established mice expressing the cytosolic Epac1-camps biosensor [19] . Interestingly, strong β 1 -AR-cAMP signals were present in both SERCA2a microdomain and bulk cytosol, while much smaller β 2 -AR-cAMP responses were detectable only in the cytosol but not with Epac1-PLN sensor targeted to the SERCA2a microdomain ( Fig. 2a–e ). Unexpectedly, the amplitudes of ISO and β 1 -AR responses measured with Epac1-PLN were higher than the signals recorded in the bulk cytosol, at ISO concentrations that saturate the responses from both sensors ( Fig. 2e ). We directly compared the sensitivities of both sensors with cAMP and found a slightly lower affinity of the targeted Epac1-PLN sensor compared with the cytosolic Epac1-camps ( Supplementary Fig. 8 ), suggesting that the actual differences between β 1 -AR responses in the SERCA2a microdomain and the cytosol might be even bigger. Using the in vitro calibration curves and our previously described protocol [18] , we converted FRET ratio values into the absolute cAMP concentrations and found about fourfold higher stimulated cAMP values in the vicinity of SERCA2a as compared with the bulk cytosol (3.9±0.4 μM in the cytosol versus 15.3±2.8 μM at SERCA2a, respectively, means±s.e., P <0.01 by one-way analysis of variance (ANOVA)). Pre-treatment of cells with the unselective PDE inhibitor 3-isobutyl-1-methylxanthin (IBMX) blunted this difference in FRET responses ( Fig. 2f ; Supplementary Fig. 9a,b ), suggesting that PDEs act to facilitate the direct receptor–microdomain communication between membrane-localized β 1 -AR and the SERCA2a-associated microdomain. Interestingly, inhibition of individual PDE families such as PDE3 or PDE4, which represent the highest PDE activities in the murine heart, did not abolish this phenomenon. However, the combined inhibition of PDE3 and PDE4 abolished the difference between the sensor responses in the two microdomains, suggesting that both PDEs in concert mediate the privileged receptor–microdomain communication ( Supplementary Fig. 9c ). These data also suggest that the targeted sensor and the new mouse model can be used to monitor the local, microdomain-specific pool of cAMP, which is different from the cAMP levels measured in the bulk cytosol. 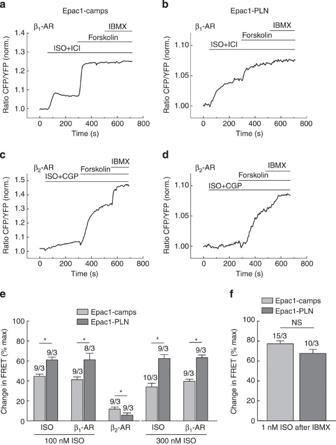Figure 2: Privileged β1-AR SERCA2a microdomain communication. (a,b) Representative FRET traces from Epac1-camps and Epac1-PLN cardiomyocytes selectively stimulated with β1-AR ligands (100 nM ISO plus 50 nM of the β2-AR blocker ICI 118551). (c,d) Representative FRET traces from Epac1-camps and Epac1-PLN myocytes after β2-AR stimulation (100 nM ISO plus 100 nM of the β1-AR blocker CGP 20712A). β2-AR has almost no effect on cAMP in the SERCA2a compartment. Subsequent maximal stimulation of adenylyl cyclase was achieved by 10 μM of forskolin, and the maximal FRET response was induced by the unselective PDE inhibitor IBMX (100 μM). (e) Quantification of the FRET experiments shown ina–d. β-AR and selective β1-AR stimulations led to significantly stronger FRET responses in the SERCA2a microdomain compared with bulk cytosol. Even at a higher ISO concentration of 300 nM, which is able to completely saturate both sensors (seeSupplementary Fig. 8C,D), there is a marked difference between the cytosol and the SERCA2a microdomain. This difference is abolished in presence of IBMX (f), suggesting the involvement of PDEs. Means±s.e., number of cells per heart is indicated above the bars. *—significant differences,P<0.05 by mixed ANOVA followed by the Waldχ2-test; NS, not significant,P>0.1 by the same test. Figure 2: Privileged β 1 -AR SERCA2a microdomain communication. ( a , b ) Representative FRET traces from Epac1-camps and Epac1-PLN cardiomyocytes selectively stimulated with β 1 -AR ligands (100 nM ISO plus 50 nM of the β 2 -AR blocker ICI 118551). ( c , d ) Representative FRET traces from Epac1-camps and Epac1-PLN myocytes after β 2 -AR stimulation (100 nM ISO plus 100 nM of the β 1 -AR blocker CGP 20712A). β 2 -AR has almost no effect on cAMP in the SERCA2a compartment. Subsequent maximal stimulation of adenylyl cyclase was achieved by 10 μM of forskolin, and the maximal FRET response was induced by the unselective PDE inhibitor IBMX (100 μM). ( e ) Quantification of the FRET experiments shown in a – d . β-AR and selective β 1 -AR stimulations led to significantly stronger FRET responses in the SERCA2a microdomain compared with bulk cytosol. Even at a higher ISO concentration of 300 nM, which is able to completely saturate both sensors (see Supplementary Fig. 8C,D ), there is a marked difference between the cytosol and the SERCA2a microdomain. This difference is abolished in presence of IBMX ( f ), suggesting the involvement of PDEs. Means±s.e., number of cells per heart is indicated above the bars. *—significant differences, P <0.05 by mixed ANOVA followed by the Wald χ 2 -test; NS, not significant, P >0.1 by the same test. Full size image Local PDE effects in hypertrophy under β-AR stimulation To directly address the hypothesis that local cAMP dynamics might be altered in cardiac disease, we used the experimental transverse aortic constriction (TAC) in vivo model to induce cardiac hypertrophy and early heart failure in both Epac1-PLN and Epac1-camps TG mice. Eight weeks after TAC, heart function was significantly decreased, to a similar extent in TG and WT littermates ( Supplementary Table 2 ), without any visible alteration of Epac1-PLN sensor localization ( Supplementary Fig. 10 ). FRET experiments in diseased cells stimulated with ISO and various PDE inhibitors revealed that after β-adrenergic stimulation, the strong effects of the PDE4 family in the bulk cytosol were significantly decreased ( Fig. 3a–c ), which was in line with a previously described reduction of the overall cytosolic PDE4 activity in severely hypertrophied and failing rat hearts [20] . In sharp contrast, the PDE4 inhibitor effects in the SERCA2a microdomains measured in the Epac1-PLN sensor-expressing CMs were unchanged after TAC. Instead, the contribution of another important PDE family PDE2 to local cAMP degradation was significantly increased ( Fig. 3d–f ). We next tested whether this change in microdomain-specific PDE-dependent effects might affect the communication between β-AR and the SERCA2a microdomain. Interestingly, the diseased cells did no longer show a difference between Epac1-camps and Epac1-PLN responses to ISO, suggesting that the receptor–microdomain communication is impaired in cardiac hypertrophy due to changes in local PDE activities ( Fig. 3g ). 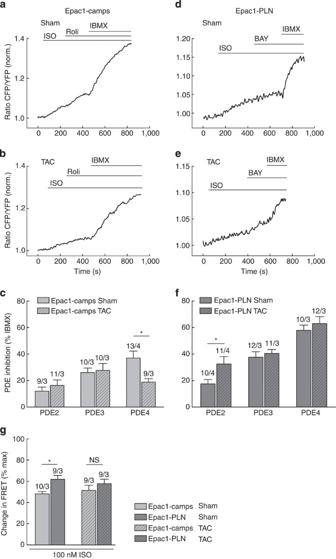Figure 3: Local PDE effects in hypertrophy under β-AR stimulation. Representative FRET traces from sham and TAC cardiomyocytes expressing Epac1-camps (a,b) or Epac1-PLN (d,e) treated with 1 nM ISO for submaximal β-AR stimulation and subsequently with the PDE4 inhibitor rolipram (Roli, 10 μM) or PDE2 inhibitor (BAY, 100 nM), respectively. In bulk cytosol, we could detect a significant decrease of PDE4 contribution after β-AR stimulation after TAC (c)—FRET values correspond to 4.2±0.8 versus 2.7±0.3 μM cytosolic cAMP measured after rolipram application, and 2.5±0.2 versus 2.5±0.3 μM after PDE2 inhibition in sham versus TAC cells, respectively. In sharp contrast, Epac1-PLN cardiomyocytes showed a significant increase of PDE2 inhibitor-induced FRET change in the TAC cells, while other PDEs were not affected (f)—FRET values correspond to 11.7±3.3 versus 23.9±3.1 μM local cAMP measured after PDE2 inhibition, and 43.8±5.8 versus 48.3±7.7 μM after PDE4 inhibition in sham versus TAC cells, respectively. PDE3 was inhibited by 10 μM cilostamide. (g) Comparison of the magnitudes of ISO responses measured with both sensors in an experiment performed as described inFig. 3e. These data argue for the impaired receptor–microdomain communication after TAC. Means±s.e., number of cells per mice is indicated above the bars. *—significant differences,Pvalues were 0.01 (inc,g), 0.04 (f) by mixed ANOVA followed by the Waldχ2-test; NS, not significant,P>0.1 by the same test. Figure 3: Local PDE effects in hypertrophy under β-AR stimulation. Representative FRET traces from sham and TAC cardiomyocytes expressing Epac1-camps ( a , b ) or Epac1-PLN ( d , e ) treated with 1 nM ISO for submaximal β-AR stimulation and subsequently with the PDE4 inhibitor rolipram (Roli, 10 μM) or PDE2 inhibitor (BAY, 100 nM), respectively. In bulk cytosol, we could detect a significant decrease of PDE4 contribution after β-AR stimulation after TAC ( c )—FRET values correspond to 4.2±0.8 versus 2.7±0.3 μM cytosolic cAMP measured after rolipram application, and 2.5±0.2 versus 2.5±0.3 μM after PDE2 inhibition in sham versus TAC cells, respectively. In sharp contrast, Epac1-PLN cardiomyocytes showed a significant increase of PDE2 inhibitor-induced FRET change in the TAC cells, while other PDEs were not affected ( f )—FRET values correspond to 11.7±3.3 versus 23.9±3.1 μM local cAMP measured after PDE2 inhibition, and 43.8±5.8 versus 48.3±7.7 μM after PDE4 inhibition in sham versus TAC cells, respectively. PDE3 was inhibited by 10 μM cilostamide. ( g ) Comparison of the magnitudes of ISO responses measured with both sensors in an experiment performed as described in Fig. 3e . These data argue for the impaired receptor–microdomain communication after TAC. Means±s.e., number of cells per mice is indicated above the bars. *—significant differences, P values were 0.01 (in c , g ), 0.04 ( f ) by mixed ANOVA followed by the Wald χ 2 -test; NS, not significant, P >0.1 by the same test. Full size image Basal cAMP levels in the SERCA2a microdomain Next, we studied which mechanisms are responsible for the control of the basal cAMP levels in the vicinity of SERCA2a and regulate the access of cytosolic cAMP pools to the microdomain. We treated Epac1-camps and Epac1-PLN cells with the selective PDE inhibitors in absence of β-adrenergic stimulation and could detect almost no FRET change in the bulk cytosol, unless multiple PDEs were inhibited with IBMX ( Fig. 4a,c,e ). In sharp contrast, clear effects of the PDE3, and especially of the PDE4 inhibitor on basal cAMP levels were detected in the SERCA2a microdomain ( Fig. 4b,d,e ). Immunoblot analysis showed that these drugs could indeed increase PLN phosphorylation when applied alone to WT cardiomyocytes ( Fig. 4f ; Supplementary Fig. 11 ), suggesting that PDE3 and 4 are involved in functional segregation of the SERCA2a microdomain from the bulk cytosol in terms of cAMP levels and their downstream effects. We next analysed whether this type of regulation might be affected in cardiac disease. Interestingly, while no significant alterations could be found after rolipram treatment in the cytosol ( Fig. 5d FRET values correspond to 1.5±0.3 versus 1.7±0.3 μM cAMP in sham versus TAC cells, respectively), Epac1-PLN cardiomyocytes showed a significant decrease of the PDE4 effect on basal cAMP levels in the SERCA2a compartment ( Fig. 5a–c ). In contrast to the FRET data, PDE activity assays in lysates from TAC cardiomyocytes did not reveal any changes in whole-cell PDE activities and PDE protein expression levels ( Supplementary Fig. 12 ). This suggests that, in contrast to chronic heart failure models of late-stage heart disease, alterations of PDE activity at the local microdomain-specific rather than at the whole-cell level occur at a milder stage of cardiac hypertrophy and may accompany transition from hypertrophy to early heart failure. These local changes can be detected only by our targeted FRET sensor approach, as in contrast to cytosolic sensors and classical biochemical techniques. Finally, immunoblot analysis of WT healthy and diseased cardiomyocytes revealed only a tendency towards decreased SERCA2a expression levels in TAC cells, which was consistent with a tendency but not with a significant difference in calcium transient kinetics ( Supplementary Fig. 13 ), suggesting that there is no impaired SERCA2a activity in our relatively mild heart failure model. 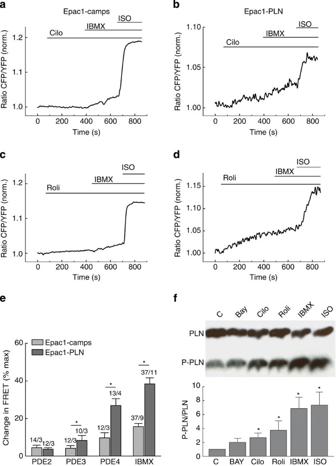Figure 4: PDE contributions to cAMP hydrolysis under basal conditions. Representative FRET traces from Epac1-camps (a,c) and Epac1-PLN (b,d) cardiomyocytes after basal PDE3 and PDE4 inhibition with cilostamide (Cilo) and rolipram (Roli), respectively. (e) Quantification of basal PDE inhibitor responses uncovered PDE3 and PDE4 as important PDE families for confining the SERCA2a microdomain from the bulk cytosol. Shown are means±s.e., number of cells per heart is indicated above the bars. *—significant differences,P<0.05 by mixed ANOVA followed by Waldχ2-test. FRET values correspond to 1.36±0.05 μM cytosolic versus 2.80±0.38 μM local cAMP measured after PDE3 inhibition, and 1.35±0.03 μM cytosolic versus 5.57±0.68 μM local cAMP after PDE4 inhibition (P<0.001 by one-way ANOVA for both PDE3- and PDE4-inhibitor-stimulated cAMP values compared in two compartments). (f) Stimulation of wildtype cardiomyocytes with the same PDE inhibitors, vehicle or ISO for 15 min leads to increased phospholamban Ser16 phosphorylation, especially after PDE4 inhibition. Means±s.e.,n=8–10 mice. *—significant differences,Pvalues compared with the control group were 0.08 (BAY), 0.02 (Cilo), 0.04 (Roli), 0.001 (IBMX) and 0.002 (ISO) by one-way ANOVA. Compound concentrations were as inFig. 3. Figure 4: PDE contributions to cAMP hydrolysis under basal conditions. Representative FRET traces from Epac1-camps ( a , c ) and Epac1-PLN ( b , d ) cardiomyocytes after basal PDE3 and PDE4 inhibition with cilostamide (Cilo) and rolipram (Roli), respectively. ( e ) Quantification of basal PDE inhibitor responses uncovered PDE3 and PDE4 as important PDE families for confining the SERCA2a microdomain from the bulk cytosol. Shown are means±s.e., number of cells per heart is indicated above the bars. *—significant differences, P <0.05 by mixed ANOVA followed by Wald χ 2 -test. FRET values correspond to 1.36±0.05 μM cytosolic versus 2.80±0.38 μM local cAMP measured after PDE3 inhibition, and 1.35±0.03 μM cytosolic versus 5.57±0.68 μM local cAMP after PDE4 inhibition ( P <0.001 by one-way ANOVA for both PDE3- and PDE4-inhibitor-stimulated cAMP values compared in two compartments). ( f ) Stimulation of wildtype cardiomyocytes with the same PDE inhibitors, vehicle or ISO for 15 min leads to increased phospholamban Ser16 phosphorylation, especially after PDE4 inhibition. Means±s.e., n =8–10 mice. *—significant differences, P values compared with the control group were 0.08 (BAY), 0.02 (Cilo), 0.04 (Roli), 0.001 (IBMX) and 0.002 (ISO) by one-way ANOVA. Compound concentrations were as in Fig. 3 . 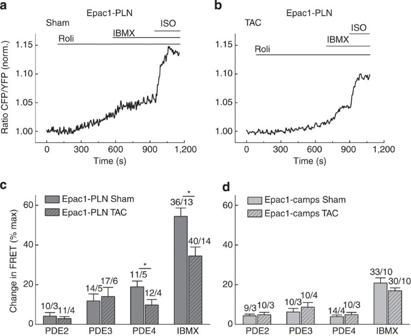Figure 5: Hypertrophy-associated changes in cAMP hydrolysis under basal conditions. Representative FRET traces from sham (a) or TAC (b) Epac1-PLN cardiomyocytes stimulated with the PDE4 inhibitor rolipram (Roli) under basal conditions before maximal stimulation with IBMX and ISO. (c) Quantification of the FRET experiments in Epac1-PLN cardiomyocytes shows a significant decrease of PDE4 contribution to basal cAMP hydrolysis in TAC cells (6.9±1.8 versus 3.4±0.9 μM cAMP measured after rolipram application, and 1.9±0.3 versus 1.5±0.5 μM after PDE2 inhibition in sham versus TAC cells, respectively). In sharp contrast, Epac1-camps cardiomyocytes do not show any change in PDE inhibitor effects (d)—FRET values correspond to 1.5±0.3 versus 1.7±0.3 μM cytosolic cAMP measured after rolipram application, and 1.4±0.5 versus 1.7±0.4 μM after PDE2 inhibition in sham versus TAC cells, respectively. Means±s.e., number of cells per mice is indicated above the bars. *—significant differences,P<0.05 by mixed ANOVA followed by the Waldχ2-test. Compound concentrations were as inFig. 3. Full size image Figure 5: Hypertrophy-associated changes in cAMP hydrolysis under basal conditions. Representative FRET traces from sham ( a ) or TAC ( b ) Epac1-PLN cardiomyocytes stimulated with the PDE4 inhibitor rolipram (Roli) under basal conditions before maximal stimulation with IBMX and ISO. ( c ) Quantification of the FRET experiments in Epac1-PLN cardiomyocytes shows a significant decrease of PDE4 contribution to basal cAMP hydrolysis in TAC cells (6.9±1.8 versus 3.4±0.9 μM cAMP measured after rolipram application, and 1.9±0.3 versus 1.5±0.5 μM after PDE2 inhibition in sham versus TAC cells, respectively). In sharp contrast, Epac1-camps cardiomyocytes do not show any change in PDE inhibitor effects ( d )—FRET values correspond to 1.5±0.3 versus 1.7±0.3 μM cytosolic cAMP measured after rolipram application, and 1.4±0.5 versus 1.7±0.4 μM after PDE2 inhibition in sham versus TAC cells, respectively. Means±s.e., number of cells per mice is indicated above the bars. *—significant differences, P <0.05 by mixed ANOVA followed by the Wald χ 2 -test. Compound concentrations were as in Fig. 3 . Full size image The importance of subcellular cAMP microdomains for cellular physiology and disease progression has been increasingly recognized and led to the development of several targeted biosensors. They have been used almost exclusively in cell lines or in neonatal cardiomyocytes [14] , rather than in more physiologically relevant adult cells or in vivo models of disease. Some other biosensors, such as the A-kinase activity reporter fused to PLN have recently been introduced into adult cardiomyocytes via adenoviral vectors to monitor local kinase activity [21] . Although we and others have successfully generated TG mice expressing some of the cytosolic FRET biosensors [19] , [22] , [23] , [24] , it remained unclear whether targeted, microdomain-specific biosensors, which act in the functionally relevant subcellular locations, are also compatible with in vivo animal models. Here, we describe the generation and validation of the first TG mouse model, which expresses a targeted cAMP biosensor designed to dissect the cAMP signalling in the vicinity of an important calcium-handling protein SERCA2a. We demonstrate that the constitutive cardiac-specific expression of such a biosensor affects neither the expression of the key players in cAMP signalling nor the normal heart physiology, apart from a measurable increase in contractility, but provides new opportunities for local cAMP imaging and studies in the context of in vivo models of cardiac disease. Our newly developed Epac1-PLN sensor showed proper co-localization with SERCA2a in TG hearts ( Fig. 1b ; Supplementary Fig. 3 ). The potential negative impact of sensor oligomerization and phosphorylation on the reliable measurements of local cAMP levels could be ruled out in experiments with cAMP-insensitive and dark Epac1-PLN mutants, as well as using a PKA inhibitor ( Supplementary Fig. 1 ). Biochemically, Epac1-PLN reflected the behaviour of endogenous PLN ( Supplementary Fig. 5 ), thereby maintaining the physiology of the SERCA2a compartment. TG mice expressing Epac1-PLN in cardiomyocytes showed a twofold overexpression of PLN without any adverse cardiac phenotype ( Supplementary Fig. 2 ), which was similar to earlier PLN TG mouse models expressing PLN only. While such models did not develop any severe phenotype apart from slightly depressed systolic function at similar amounts of overexpression [25] , [26] , the contractile function in Epac1-PLN mice was slightly but clearly increased ( Supplementary Table 1 ). This discrepancy might be due to the compensatory upregulation of SERCA2a protein expression in our Epac1-PLN mouse model or to the intrinsic properties of the sensor molecule, but not of the overexpressed PLN ( Supplementary Fig. 4 ). Another possibility is that a slight decrease in heart rate ( Supplementary Tables 1 and 2 ) is responsible for a compensatory increase of contractility, although the mechanism that lowers the heart rate in TG mice is unclear. Epac1-PLN mice provide a valuable source of primary cells to study previously established and potentially new mechanisms of cAMP compartmentation in an optimal physiological and pathophysiological context. Despite a reduced dynamic range of the sensor ( ∼ 10% maximal measured FRET change of Epac1-PLN compared with ∼ 30–40% for the cytosolic responses measured with Epac1-camps, see Supplementary Fig. 1c and Figs 2 , 3 , 4 ), the new Epac1-PLN sensor had a sufficient signal-to-noise ratio and sensitivity to resolve local cAMP responses in healthy and diseased cardiomyocytes (as judged by the quality of traces and data summary in Figs 2 , 3 , 4 , 5 ). Since the confounding factors such as intermolecular FRET due to pentamer formation or PKA-dependent effects could be ruled out (see Supplementary Fig. 1 ), the observed reduction of the dynamics range might be due to other reasons. Comparison of corrected non-normalized acceptor/donor ratios between Epac1-camps- and Epac1-PLN-expressing cells ( Supplementary Fig. 14 ) showed that these ratios were comparable at the basal state. However, Epac1-PLN ratio values were higher in the fully stimulated sensor. This suggests that in the targeted sensor, the end-point ratio in the bound state might be altered, for example, due to reduced conformational change in the sensor. An increase in local cAMP levels in the SERCA2a microdomain was not detectable after β 2 -AR stimulation, which is in line with previous studies showing no effect of β 2 -AR-cAMP on PLN phosphorylation [27] and its stringent compartmentation at the T-tubular membranes [28] , [29] . However, the relatively small β 2 -AR-cAMP signals are potentially difficult to resolve, especially using the less sensitive Epac1-PLN sensor, which is certainly a limitation of our study. Strikingly, full stimulation of β 1 -AR at equilibrium led to much higher cAMP levels in the SERCA2a microdomain compared with bulk cytosol ( Fig. 2 ). This indicates that a specific compartment deep inside the cell might have a privileged access to the pool of cAMP formed after stimulation of a particular membrane receptor, thereby sensing higher second messenger levels compared with the bulk cytosol due to a PDE-dependent ‘channelling’ of cAMP from the membrane to the microdomain. It has previously been shown in HEK293 cells after prostaglandin E 1 stimulation that PDEs act as local sinks that drain cAMP gradients towards specific contiguous subcellular compartments such as the nucleus [30] . This mechanism allows coexistence of multiple microdomains with various cAMP concentrations independently of their distance from the place of cAMP synthesis, which we now show to occur in physiologically most relevant adult cardiomyocytes and to be regulated by the joint action of PDE3 and PDE4 ( Supplementary Fig. 9c ). In this study, we use our newly developed mouse model to provide the first insights into alterations of local cAMP dynamics at SERCA2a in cardiac hypertrophy at the transition to early heart failure. Despite TG sensor expression and slightly but clearly increased cardiac contractility, Epac1-PLN animals, similar to WT mice, developed pronounced cardiac hypertrophy after TAC ( Supplementary Table 2 ), suggesting that the TG model can be used to study local cAMP signalling in context of disease. We could show that after β-AR stimulation, PDE4 contribution in the cytosol was significantly decreased in hypertrophied cardiomyocytes ( Fig. 3c ), which is consistent with previous results from rats with severe cardiac hypertrophy where the activities of both PDE4A and PDE4B were significantly reduced [20] . Interestingly, in our experimental model, the whole-cell PDE activity measured by the same assay was not yet decreased ( Supplementary Fig. 12 ), suggesting that at this time point of disease progression, local microdomain-specific rather than whole-cell changes in PDE activity and possibly also localization [31] might take place. The strength of our approach is that, using targeted biosensors and in vivo models, we can resolve local changes of cAMP at an early stage of disease progression before they become apparent using classical techniques, and at a time point that might be potentially attractive for early therapeutic interventions. In sharp contrast to PDE4, PDE2 inhibition led to a significantly higher FRET change in the SERCA2a compartment after TAC ( Fig. 3f ). Recently, we showed marked upregulation of PDE2 at the whole-cell level in various chronic cardiac disease models and a significant decrease of PKA-mediated PLN phosphorylation in PDE2-overexpressing cardiomyocytes after ISO stimulation [32] . These results are consistent with our findings that PDE2 inhibition in diseased Epac1-PLN cardiomyocytes induced a FRET change exclusively upon ISO stimulation rather than under basal conditions. This might indicate a mechanism by which PDE2 upregulation protects the heart and especially the SERCA2a compartment from cAMP overflow due to the decreased PDE4 contribution in the cytosol of diseased cardiomyocytes. Strikingly, the privileged signal communication between the β 1 -AR and SERCA2a was impaired in hypertrophy ( Fig. 3g ). This argues for the fact that the disease-associated remodelling of PDE effects in various microdomains leads to impressive changes of cAMP compartmentation ( Fig. 6 ), which might have far-reaching functional consequences. 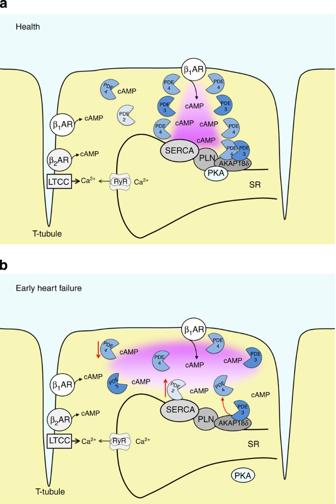Figure 6: Schematics showing proposed changes of local cAMP signalling in disease. (a) In healthy cardiomyocytes, β1- but not β2-AR-cAMP pools reach the SERCA2a microdomain, whereby there is a privileged communication between β1-AR and the microdomain through a dynamic ‘channel’ formed by the orchestrated action of PDE3/4. The access of the cytosolic cAMP to SERCA2a in absence of receptor stimulation is controlled by the local pools of PDE3 and PDE4. (b) In early heart failure, the SERCA2a-associated (at basal state) and the cytosolic (after β-adrenergic stimulation) PDE4 effects are lost, while the local PDE2-dependent effects are increased, leading to a loss of effective receptor–microdomain communication. Figure 6: Schematics showing proposed changes of local cAMP signalling in disease. ( a ) In healthy cardiomyocytes, β 1 - but not β 2 -AR-cAMP pools reach the SERCA2a microdomain, whereby there is a privileged communication between β 1 -AR and the microdomain through a dynamic ‘channel’ formed by the orchestrated action of PDE3/4. The access of the cytosolic cAMP to SERCA2a in absence of receptor stimulation is controlled by the local pools of PDE3 and PDE4. ( b ) In early heart failure, the SERCA2a-associated (at basal state) and the cytosolic (after β-adrenergic stimulation) PDE4 effects are lost, while the local PDE2-dependent effects are increased, leading to a loss of effective receptor–microdomain communication. Full size image Interestingly, under basal conditions without β-AR stimulation, PDE3 and especially PDE4 play a critical role in confining the SERCA2a microdomain from the bulk cytosol to limit the basal PLN phosphorylation ( Fig. 4 ). Using a targeted PKA activity reporter AKAR3 fused to PLN and expressed in neonatal rat cardiomyocytes, it was recently shown that under basal conditions, PKA activity in this microdomain is also lower and controlled by PDE4 (ref. 17 ). Furthermore, using PDE3A and PDE3B null mice, it was demonstrated that PDE3A functionally interacts with SERCA2a, thereby regulating basal myocardial contractility [33] . Another study in PDE4D null mice could detect PDE4D as a critical regulator of baseline SR-Ca 2+ release [34] . Together with these findings, our live cell imaging data indicate that PDE3 and PDE4 are both involved in the regulation of basal local cAMP dynamics in the SERCA2a microdomain and contractility of healthy hearts. However, in early heart failure, the local PDE4, but not PDE3, effect responsible for confining the SERCA2a microdomain under basal conditions is markedly decreased ( Fig. 5 ). Interestingly, the SERCA2a function at this stage of disease is not yet significantly impaired, as demonstrated by calcium transient measurements ( Supplementary Fig. 13 ). It might be that the local PDE4 downregulation in cardiac hypertrophy represents a protective mechanism to initially compensate for the loss of SERCA2a function before the heart will be transitioning towards a functionally decompensated state, where the decrease of PDE4 activity can no longer compensate for the loss of SERCA2a function. In addition, the possible loss of local PKA activity in the microdomain [35] might impair the regulatory feedback loops engaged by PKA-dependent PDE4 phosphorylation. In general, it is relatively challenging to directly compare FRET responses side-by-side between two different biosensors (one cytosolic and another one localized) with different dynamic ranges and cAMP affinities. Therefore, this represents an important limitation of our study. However, a reliable strategy to overcome this problem is to perform accurate calibration of both sensors and to recalculate the FRET ratio data into absolute cAMP concentrations or equivalents of the generalized forskolin responses [18] , [36] . We chose the first option and provided the accurately calculated cAMP values for all key experiments, which directly compare responses from both sensors to support our conclusions (see Figs 2e and 4e ). Another limitation is the different sensor cAMP response kinetics due to different affinities, which is intrinsic to the molecular sensor. Therefore, we compared the FRET data only at the apparent equilibrium of any response and did not directly compare signal kinetics. In the future, through advanced molecular design and optimization of targeted sensors, ideally similar cAMP affinities and dynamics range with and without targeting to various subcellular compartments can be achieved. In summary, we developed TG mice for direct real-time monitoring of cAMP dynamics in the SERCA2a microdomain, and demonstrated biocompatibility of a targeted FRET biosensor as well as its usefulness in the context of an in vivo disease model. We further established the privileged receptor–microdomain communication as a PDE3/4-dependent mechanism of cAMP compartmentation, which is affected in disease, thereby impairing β-AR-cAMP signalling to SERCA. We believe that our model should offer exciting new possibilities to study microdomain-specific signalling in a more physiological setting of healthy and diseased organisms. Development of Epac1-PLN biosensor DNA sequence of the cytosolic cAMP sensor Epac1-camps [16] without the stop codon was fused to the full-length or N-terminally truncated human PLN as shown in Supplementary Fig. 1 . The resulting construct was subcloned via KpnI/XhoI restriction sites into a vector containing the α-MHC promoter, which was used for generation of TG mice [28] . In addition to the functional Epac1-PLN construct, the cAMP-insensitive mutant was generated by exchanging the cAMP-binding domain sequence in this sensor with a sequence containing the R279E point mutation [18] . To generate dark CFP and dark YFP constructs, the following mutations were introduced into Epac1-PLN sequence via site-directed mutagenesis: W66G in CFP, and Y66G in YFP. Generation of TG mice The α-MHC-based vector encoding Epac1-PLN was linearized using NotI, purified and used for pronuclear injection of FVB/N mice [37] . Founder mice and their resulting heterozygote offspring were genotyped by a standard PCR using the primers: 5′-TGACAGACAGATCCCTCCTAT-3′ and 5′-CATGGCGGACTTGAAGAAGT-3′, resulting in a ∼ 340-bp fragment on a gel. Positive founder mice were mated with WT FVB/NRj animals (obtained from Janvier Labs, Saint Berthevin, France) to produce heterozygous offspring. Cardiomyocyte isolation Adult ventricular cardiomyocytes were isolated via the Langendorff perfusion [18] , [38] . Mice were euthanized and the hearts were quickly transferred into a chamber filled with ice-cold PBS (Biochrom) where the aorta was connected to a 21G cannula. The heart was Langendorff perfused at 37 °C with Ca 2+ -free perfusion buffer (in mM: NaCl 113, KCl 4.7, KH 2 PO 4 0.6, Na 2 HPO 4 × 2H 2 O 0.6, MgSO 4 × 7H 2 O 1.2, NaHCO 3 12, KHCO 3 10, HEPES 10, Taurine 30, 2,3-butanedione-monoxime 10, glucose 5.5, pH 7.4) for 3 min followed by 30 ml digestion buffer containing liberase DH (0.04 mg ml −1 , Roche), trypsin (0.025%, Gibco) and CaCl 2 12.5 μM. Afterwards, the atria were carefully excised and discarded, whereas the digested ventricles were dissected for 30 s in 2.5 ml digestion buffer. To stop the digestion, 2.5 ml Stop buffer I (perfusion buffer containing 1% BSA (Sigma, Deisenhofen, Germany) and 50 μM CaCl 2 ) were added to the cell suspension, which was then homogenized for 3 min using a 1-ml syringe without a needle. Ten minutes after sedimentation, the cardiomyocyte pellet was transferred into Stop buffer II (perfusion buffer containing 0.5% BSA and 37.5 μM CaCl 2 ) for gradual recalcification up to 1 μM of calcium. The cardiomyocytes were plated onto round laminin (Sigma)-coated coverslides (24 mm, Thermo Scientific) and incubated at 37 °C and 5% CO 2 until use. For immunoblot analysis, cardiomyocyte isolation was performed in the same way, but the Stop buffer II did not contain BSA. FRET measurements and data analysis Laminin-coated coverslides with isolated cardiomyocytes were mounted in the custom-made imaging chamber (similar to Attofluor chamber, Life Science Technologies). The cells were washed once with 300 μl of FRET buffer (in mM: 144 NaCl, 5.4 KCl, 1 MgCl 2 , 1 CaCl 2 , 10 HEPES, pH 7.3), and 300 μl of the same buffer were added to the chamber. FRET measurements were performed using an inverted fluorescent microscope (Nikon T i ) and ImageJ software [39] . The FRET donor CFP was excited at 440 nm using a CoolLED light source. Cardiomyocytes with optimal sensor expression were selected using live fluorescent light, which was immediately switched off after finding an appropriate cell to avoid photobleaching of the FRET sensor. The exposure time was usually 10 ms, which led to good signal-to-noise ratio, and images in CFP and YFP emission channels were acquired every 5 s. Three hundred μl of the desired compound solution (in FRET buffer) were transferred into the chamber as soon as the FRET ratio reached a stable baseline. FRET imaging data were analysed offline using Origin 8.5 software. The single CFP and YFP intensities from each experiment were measured using ImageJ and copy-pasted into an Excel or Origin spreadsheet to calculate the corrected FRET ratio. We corrected for the bleedthrough of the donor fluorescence (CFP) into the acceptor (YFP) channel, in our case ratio=(YFP−0.63 × CFP)/CFP. Transverse aortic constriction (TAC) All animal experiments were performed in accordance with the guidelines of the University Medical Centre Göttingen and the guidelines defined by the state of Lower Saxony. Female mice aged 8–12 weeks were randomized into sham or TAC groups. Mice were anesthetized using 2% isoflurane in 100% oxygen. A suprasternal incision was made, and the aortic arch was visualized using a binocular operating stereoscope (Olympus). TAC interventions used a spacer-defined (26-gauge) constriction fixed by a 6-0 polyviolene suture between the first and second trunk of the aortic arch [40] . For sham, the aorta was exposed as for TAC but not constricted. Three days post TAC intervention, Doppler velocity was measured by a 20-MHz probe to quantify the pressure gradient across the TAC region or after the sham procedure by transthoracic echocardiography (VisualSonics Vevo 2100; Toronto, Canada). Three days before and during 1 week after surgery, mice received analgesic therapy with metamizole. Eight weeks after surgery, mice were analysed by echocardiography, and hearts were harvested for ventricular cardiomyocyte isolation or histology. Quantitative real-time PCR Heart tissue RNA was isolated using the RNeasy purification Kit (Qiagen), and subsequent cDNA synthesis was performed using the iScript cDNA Synthesis Kit (Bio-Rad). Standard genes were amplified using 1:10 dilution of WT cDNA and GoTaq Polymerase (Promega) with the following PCR protocol. Primers used for GAPDH were 5′-GTTGTCTCCTGCGACTT-3′ and 5′-GGTCCAGGGTTTCTTACT-3′, for PLN: 5′-CAATACCTCACTCGCTC-3′ and 5′-ATGATGCAGATCAGCAG-3′. Standards were purified using the Qiagen PCR Kit and eluted in 30 μl of buffer EB. Standard purity was assured by agarose gel electrophoresis of 2 μl standard eluate. Standard dilutions ranging from 100 pg μl −1 to 1 ag μl −1 were prepared in RNase-free H 2 O. Quantitative real-time PCR was conducted using the SYBR Green Super Mix for iQ (Quanta Bisosciences) and the icycler (Bio-Rad) according to the following protocol: Data were analysed using Bio-Rad iQ5 software, and PLN mRNA levels were normalized to GAPDH mRNA levels of the same cDNA sample. Gene arrays Cardiomyocyte RNA from total of five individual WT and five TG mice was isolated using the RNeasy purification Kit (Qiagen) according to the manufacturer protocol, diluted with RNAse-free water to 200–350 ng μl −1 and submitted for the Illumina gene array analysis to the Göttingen transcriptome analysis laboratory (TAL). Fractionation and immunoblot analysis For fractionation analysis, whole hearts were perfused with ice-cold PBS (Biochrom) until blood free and then shock frozen. Heart tissue was processed using the Qproteome Cell Compartment Kit (Qiagen); cytosolic and membrane fractions were subjected to 10–15% SDS–polyacrylamide gel electrophoresis and to immunoblotting using anti-PLN A-1 (Badrilla, 1:2,500), anti-SERCA2a (Badrilla 1:5,000), anti-GFP (Santa Cruz (Santa Cruz, CA), 1:500) and anti-GAPDH (HyTest, 1:36,000) antibodies according to the manufacturer’s protocols. To analyse PLN phosphorylation under basal and various stimulated conditions, freshly isolated cardiomyocytes sedimented in Stop buffer II without BSA were incubated either with vehicle, 100 nM ISO, 100 nM BAY 60-7550, 10 μM cilostamide, 10 μM rolipram or 100 μM IBMX for 15 min at 37 °C. Cell pellets were shock frozen, and homogenized proteins were quantified using BCA Protein Assay (Pierce). Samples were boiled at 95 °C for 5 min to disrupt PLN pentamers. Ten to twenty μg of total protein were subjected to 15% SDS–polyacrylamide gel electrophoresis and immunoblotting using the anti-P-Ser16 phospholamban (Badrilla 1:5,000) and anti-PLN A-1 antibodies (Badrilla). To compare protein levels between WT and TG cells, PKA RI and RII subunits were probed with BD Biosciences antibodies (1:500). PDE2A and PDE4D8 expression was analysed using anti-PDE2A (Fabgennix, 1:750) and a custom-made PDE4D8 antibody (1:2,000, kindly provided by Marco Conti), respectively. TAC and sham cardiomyocyte lysates were immunoblotted using anti-PDE2A (Fabgennix, 1:750), anti-PDE4D (Santa Cruz, 1:200) and anti-calsequestrin (Thermo Scientific, 1:10,000) antibodies according to the manufacturer’s protocols. Band densitometry analysis was performed using ImageJ software. PDE activity assay Freshly isolated cardiomyocytes were lysed and processed for in vitro measurement of cAMP-PDE hydrolysing activity following the standard method by Thompson and Appleman in presence of 1 μM cAMP as a substrate [41] . In brief, contributions of individual PDE families were calculated from the effects of 100 nM BAY (PDE2), 10 μM cilostamide (PDE3), 10 μM rolipram (PDE4) and 100 μM IBMX (unselective inhibitor). Isolated cardiomyocytes sedimented in Stop buffer I (see cardiomyocyte isolation) were washed with wash buffer (40 mM Tris-Cl, pH 8.0) and lysed in 500 μl of homogenization buffer (wash buffer containing 10 μmol l −1 MgCl 2 plus protease- and phosphatase inhibitors (Roche)). Proteins were quantified using the BCA Protein Assay (Pierce). Thirty μg protein were set to a total volume of 200 μl homogenization buffer containing inhibitors. For maximal cAMP breakdown, each sample was incubated with 200 μl reaction buffer (wash buffer containing: 10 mM MgCl 2 , 10 mM 2-mercaptoethanol, 2 μM cAMP (Sigma), 1.5 mg ml −1 BSA and 0.1 μCi [ 3 H]-cAMP (American Radiolabeled Chemicals Inc.) for 10 min at 33 °C. Reaction was terminated by adding 200 μl stop solution (wash buffer containing 15 mM EDTA, pH 8.0) and heat inactivation for 1 min at 95 °C. The samples were incubated with 50 μg of Crotalus atrox snake venom (Sigma) for 20 min at 33 °C to hydrolyse the 5′-AMP. The samples were loaded onto columns containing 50 mg AG1-X8 resin (Bio-Rad) for anion-exchange chromatography to separate the adenosine. Quantification was performed by scintillation counting. Histology, morphometric analysis and echocardiography Echocardiography [42] of WT and TG Epac1-PLN mice was performed at the age of 3 and 6 months using the Vevo 2100 system (VisualSonics) equipped with a 30-Hz transducer (MS-400 MicroScan Transducer). For histology and morphometric analysis, WT and TG hearts were harvested, perfused with PBS until blood free and fixed in 4% Roti Histofix (Roth) at 4 °C overnight. The fixed hearts were embedded in paraffin, and 5 μm heart cross-sections were generated by Microtom (Leica RM 2165). For the following applications, paraffin cross-sections were dewaxed and rehydrated in xylol (20 min twice) with four subsequent decreasing ethanol series (5 min each step). The haematoxylin–eosin stain of WT and TG heart sections was performed in the pathology department of the University Medical Center Göttingen using a standard automated procedure. Cell nuclei were stained thrice with haematoxylin (2 min each), and after 2 min washing, the cytosol was stained twice using eosin (2 min each). After rehydration and mounting, heart sections were analysed using a Stemi 2000-C microscope binocular with associated AxioCam ICc1 and AxioVision software (Carl Zeiss MicroImaging, Jena, Germany). To determine cardiomyocyte dimensions, WT and TG heart cross-sections were incubated with wheat germ agglutinin (75 μg μl −1 , Sigma) for 30 min in the dark, washed with PBS thrice, mounted and observed under a Axiovert 200 microscope (Carl Zeiss MicroImaging). AxioVision software (Carl Zeiss MicroImaging) was used for image acquisition. The cell diameters of 100 cells from each heart section were measured and analysed using ImageJ. Immunostaining Immunostaining of TG Epac1-PLN heart cross-sections was performed after heat-induced epitope retrieval in citrate buffer (Dako, dilution 1:10). We used primary antibodies for SERCA2a (Badrilla, dilution 1:100), and GFP (Santa Cruz, dilution 1:500) to detect Epac1-PLN. The secondary antibodies were Alexa Fluor 633 (Invitrogen, dilution 1:300) and Alexa Fluor 514 (Invitrogen, dilution 1:500), respectively. After rehydration, the stained heart sections were mounted, and image acquisition was performed using confocal microscopy. Confocal microscopy Confocal microscopy was performed using Zeiss LSM 710 NLO microscope (Carl Zeiss MicroImaging) equipped with a Plan-Apochromat × 63/1.40 oil-immersion objective. Images were acquired for Alexa Fluor 514 (514 nm argon ion laser excitation) and Alexa Fluor 633 (633 nm diode laser excitation). ZEN 2010 software (Zeiss) was used for image analysis. For Supplementary Fig. 1d , CFP and YFP were excited with 405-nm diode and 514-nm argon ion lasers, respectively. Calcium transients of single cardiomyocytes Freshly isolated cardiomyocytes were plated onto laminin-coated glass coverslides and incubated with 1 μM Fura2-AM or Fluo3-AM (Life Science Technologies) for 15 min at 37 °C in Tyrode solution (in mM: KCl 1, NaCl 149, MgCl 2 1, HEPES 5, Glucose 10, CaCl 2 1, pH=7.54). After washing the cells thrice with Tyrode solution, myocytes were field stimulated at 1 Hz until steady state was achieved, and then calcium transients were recorded for 60 s using the epifluorescence system. F / F 0 values were calculated from the ratios of 510 nm emission light measured at 340 and 380 nm excitations in case of Fura2, or the calcium transient decays were determined from Fluo3 fluorescence traces. For calcium transient decays, the time constant tau ( τ ) was calculated using IonWizard software. Chemicals IBMX was from AppliChem. BAY 60-7550 was from Santa Cruz. ISO, rolipram, forskolin, cilostamide, ICI 118551, CGP 20712A, 8-methoxymethyl-3-isobutyl-1-methylxanthine, and all other substances were from Sigma. Statistics Echocardiographic, morphometric, real-time PCR and FRET data were analysed using the Origin Pro 8.5 software (OriginLab Corporation, Northhampton, MA). Normal distribution was tested by the Kolmogorov–Smirnov test, and differences between the groups were analysed using mixed ANOVA followed by Wald χ 2 -test, one-way ANOVA for simple two-group comparison or Kruskal–Wallis ANOVA, as appropriate, at the significance level of 0.05. Sample sizes were 3–6 mice and 8–17 measured cells. No sample exclusion was performed, except for TAC mice that were not studied if the pressure gradients did not reach 50 mm Hg (standard cutoff for the development of reliable pressure-overload-induced hypertrophy). Acccession codes: Microarray data have been deposited in Gene Expression Omnibus under accession code GSE65651 . How to cite this article: Sprenger, J. U. et al. In vivo model with targeted cAMP biosensor reveals changes in receptor–microdomain communication in cardiac disease. Nat. Commun. 6:6965 doi: 10.1038/ncomms7965 (2015).